The oncogenic microRNA miR-21 promotes regulated necrosis in mice MicroRNAs (miRNAs) regulate apoptosis, yet their role in regulated necrosis remains unknown. miR-21 is overexpressed in nearly all human cancer types and its role as an oncogene is suggested to largely depend on its anti-apoptotic action. Here we show that miR-21 is overexpressed in a murine model of acute pancreatitis, a pathologic condition involving RIP3-dependent regulated necrosis (necroptosis). Therefore, we investigate the role of miR-21 in acute pancreatitis injury and necroptosis. miR-21 deficiency protects against caerulein- or L -arginine-induced acute pancreatitis in mice. miR-21 inhibition using locked-nucleic-acid-modified oligonucleotide effectively reduces pancreatitis severity. miR-21 deletion is also protective in tumour necrosis factor-induced systemic inflammatory response syndrome. These data suggest that miRNAs are critical participants in necroptosis and miR-21 enhances cellular necrosis by negatively regulating tumour suppressor genes associated with the death-receptor-mediated intrinsic apoptosis pathway, and could be a therapeutic target for preventing pathologic necrosis. Recent advances in the understanding of the fundamental biology of cellular death have led to the identification of two distinct, but interrelated, forms of programmed cell death—apoptosis and regulated necrosis [1] . Apoptosis involves the engagement of intrinsic or extrinsic pathways that activate caspase proteases. Morphologically, necrotic cells differ significantly from apoptotic cells. For example, necrotic cells exhibit translucent cytoplasm, swelling of organelles and disruption of the plasma membrane with release of endogenous molecules such as lactate dehydrogenases (LDHs), ATP, ions and DNA that directly trigger a pro-inflammatory response. On the other hand, cells undergoing apoptosis display chromatin aggregation, nuclear and cytoplasmic condensation, and partitioning of cytoplasm and nucleus into membrane-bound vesicles. Moreover, unlike necrosis, apoptosis is not usually associated with tissue inflammation, because phagocytic cells efficiently clear apoptotic cells. Once regarded as an unscheduled and unregulated cell death induced by nutrient deprivation and traumatic or toxic injury, necrotic cell death in some contexts has been found to be a regulated process driven by defined molecular pathways [2] . Among many forms of regulated necrosis, necrotic cell death that depends on receptor-interacting protein 3 (RIP3, also known as RIPK3) is termed as necroptosis, a cellular process integrated with the extrinsic apoptosis pathway. Extrinsic apoptosis is regulated by death receptors such as tumour necrosis factor (TNF)-α receptor 1 (TNFR1) and CD95 that activate cell death pathways when engaged by their cognate ligands such as TNF-α and FasL (also known as CD95L). This extrinsic death pathway is mediated by the adaptor protein Fas-associated protein with a death domain (FADD), which couples the receptor-generated signals to the death-executing protease enzyme, caspase-8. Activation of caspase-8 triggers downstream effector caspases to initiate the classical apoptosis cascade. In contrast, TNFR-mediated initiation of necroptosis requires the kinase activity of RIP1 (also known as RIPK1) and RIP3, and its execution involves the active disintegration of mitochondrial membranes [1] , [3] , [4] . RIP1 and RIP3 are components of the necrosome, and caspase-8 can directly cleave and inactivate both kinases to negatively regulate necroptosis induced by TNF-α [5] , [6] , [7] . On pharmacological inhibition of caspase, RIP1 and RIP3 are phosphorylated to trigger necroptosis. The interplay of apoptosis and necroptosis is further demonstrated in recent mouse genetic experiments showing that ablation of RIP3 or RIP1 protects caspase-8-null or FADD-null mice from embryonic lethality [6] , [7] , [8] , [9] . Necroptosis is associated with several pathologic conditions, including acute pancreatitis, ischaemia–reperfusion injury, neurodegeneration and infection [1] . In an experimental model of acute pancreatitis, mice treated with supramaximal doses of caerulein predominantly display necrosis with little apoptosis and the degree of necrosis correlates with injury severity [10] . Embryonic fibroblasts from RIP3-null mice have been found to be resistant to necrosis and RIP3-null mice are devoid of inflammation-inflicted tissue damage in caerulein-induced acute pancreatitis, indicating RIPs are important in necroptosis [3] . Over 1,000 human microRNAs (miRNAs) have been discovered so far [11] and they are predicted to target up to 92% of all human genes [12] . The role of miRNAs in cell death, in particular in apoptosis, has been extensively investigated. miR-21 is the most studied miRNA and data from various transgenic and/or deficient mouse models of miR-21 indicate that miR-21 exerts its oncogenic function predominantly through inhibiting cellular apoptosis [13] , [14] , [15] . However, the role of miR-21 or any other miRNA in necroptosis remains completely unknown. In the present study, we report that miR-21 is overexpressed in a murine model of acute pancreatitis, a condition characterized by cellular necrosis. Genetic ablation of miR-21 in mice protects against caerulein- or L -arginine ( L -Arg)-induced acute pancreatitis. Pharmacological miR-21 inhibition significantly reduces pancreatitis severity in wild-type (WT) mice. In addition, miR-21 deficiency is protective in TNF-induced tissue injury. Our results suggest that miR-21 promotes TNF-α-induced necroptosis and indicate miR-21 is a potential therapeutic target for drug development against diseases associated with cellular necrosis. Role of miR-21 in caerulein-induced acute pancreatitis To study the role of miR-21 in acute pancreatitis, we first measured the expression of miR-21 in WT mice treated with PBS-formulated caerulein, using quantitative real-time PCR. We found that compared with untreated or PBS-treated controls, the ΔC t values of miR-21 normalized to a reference RNA (snoRNA292) were significantly lower ( P =0.003; Fig. 1a ) in the pancreas from mice at day 1 after the last caerulein injection, when the severity of acute pancreatitis was at its peak [16] . The difference in ΔC t values represents a >16-fold upregulation of miR-21 (using either mean or median values). Correspondingly, at day 3 and day 7 post treatment, miR-21 expression was reduced ( Fig. 1a ). 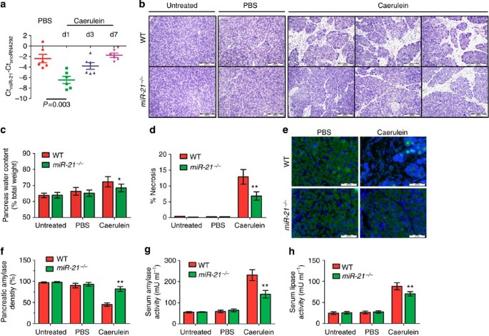Figure 1: Response of WT andmiR-21−/−mice to caerulein. (a) Expression of miR-21 during caerulein-induced pancreatitis in WT mice (n=6 per group). Pancreatic tissue was harvested at day 1 (d1), day 3 (d3) and day 7 (d7) after the last caerulein or PBS (control) injection. (b) Representative histological sections of mouse pancreata stained with haematoxylin from caerulein-treated WT andmiR-21−/−mice. Scale bars, 200 μm. (c) Water content of the pancreas from caerulein-treated WT andmiR-21−/−mice at d1 (n=5 per group) after the last dose of caerulein. (d) Percentage of necrotic cells in pancreata from WT andmiR-21−/−mice. (e) Immunofluorescence staining for amylase at day 1 after the last caerulein injection. Scale bars, 100 μm. (f) Morphometric analysis of amylase density (percentage of amylase-positive areas within five microscopy fields per slide per animal; five animals per group). (g) Serum amylase activity in WT andmiR-21−/−mice (n=12 per group) 6 h after the last caerulein injection. (h) Serum lipase activity in WT andmiR-21−/−mice (n=12 per group) at 6 h after the last caerulein injection. Values are mean±s.d. (n=6). **P<0.01 indicates a significant difference between WT andmiR-21−/−mice treated with caerulein (one-way analysis of variance (ANOVA) inaand two-way ANOVA in others). Figure 1: Response of WT and miR-21 −/− mice to caerulein. ( a ) Expression of miR-21 during caerulein-induced pancreatitis in WT mice ( n =6 per group). Pancreatic tissue was harvested at day 1 (d1), day 3 (d3) and day 7 (d7) after the last caerulein or PBS (control) injection. ( b ) Representative histological sections of mouse pancreata stained with haematoxylin from caerulein-treated WT and miR-21 −/− mice. Scale bars, 200 μm. ( c ) Water content of the pancreas from caerulein-treated WT and miR-21 −/− mice at d1 ( n =5 per group) after the last dose of caerulein. ( d ) Percentage of necrotic cells in pancreata from WT and miR-21 −/− mice. ( e ) Immunofluorescence staining for amylase at day 1 after the last caerulein injection. Scale bars, 100 μm. ( f ) Morphometric analysis of amylase density (percentage of amylase-positive areas within five microscopy fields per slide per animal; five animals per group). ( g ) Serum amylase activity in WT and miR-21 −/− mice ( n =12 per group) 6 h after the last caerulein injection. ( h ) Serum lipase activity in WT and miR-21 −/− mice ( n =12 per group) at 6 h after the last caerulein injection. Values are mean±s.d. ( n =6). ** P <0.01 indicates a significant difference between WT and miR-21 −/− mice treated with caerulein (one-way analysis of variance (ANOVA) in a and two-way ANOVA in others). Full size image Next, we evaluated the changes in pancreatic histology at 1, 3 and 7 days after the last caerulein injection. In WT mice, extensive acinar cell injury and necrosis in pancreatic tissue were found at day 1 ( Fig. 1b ). At day 3 the pancreatic tissue morphology was in the process of recovering, and at day 7 it appeared normal ( Supplementary Fig. 1a,b ). This agrees with existing knowledge that pancreatic regeneration after acute pancreatitis induced by caerulein is largely completed within a week, when the pancreas histology is similar to healthy untreated controls [16] . In contrast, miR-21 −/− mice at day 1 had dramatically less pancreatic injury ( Fig. 1b ). Furthermore, histological analyses showed reduced pancreatic edema and acinar cell necrosis in miR-21 −/− mice ( Fig. 1c,d ). Pancreatic regeneration at days 3 and 7 in miR-21 −/− mice, however, was similar to that in WT mice ( Supplementary Fig. 1a,b ), probably because regeneration after caerulein-induced injury is partially completed by day 3, and by day 7 it is completed in both WT and miR-21 −/− mice. We performed immunofluorescence staining for amylase in the pancreata and confirmed a substantial loss of exocrine cells in WT mice, but not in miR-21 −/− mice, at day 1 post treatment ( Fig. 1e,f ). Elevated amylase and lipase activity in the serum is a hallmark of acute pancreatitis in both humans and mice [17] , [18] , [19] . Compared with WT mice, both serum amylase and lipase activity in miR-21 −/− mice were significantly lower 6 h after the final dose of caerulein ( Fig. 1g,h ). Taken together, these results suggest that miR-21 deficiency protects against acute pancreatitis induced by caerulein in mice. In addition to acinar cell injury, another feature of acute pancreatitis is damage to distal organs such as the lung. As shown in Supplementary Fig. 2 , lung injury in WT mice manifested as thickened alveolar membranes and neutrophil sequestration as reflected by higher myeloperoxidase (MPO) enzyme activity. In contrast, alveolar membrane thickening and MPO activity were markedly lower in miR-21 −/− mice treated with caerulein compared with WT mice. These observations indicate that genetic ablation of miR-21 reduces the severity of lung injury following caerulein-induced pancreatitis. Regulation of inflammatory cell infiltrate by miR-21 Monocyte-derived macrophages are known to infiltrate the pancreata during acute pancreatitis and to act as inflammatory mediators that participate in the pathophysiology of pancreatitis [20] , [21] . Thus, we determined whether miR-21 deletion reduces inflammatory cell infiltration. On caerulein treatment, CD11b-positive cells (that is, monocytes and macrophages) rapidly migrated to the injured pancreata of WT mice starting day 1 after caerulein treatment ( Fig. 2a,b ); however, in miR-21 −/− mice the number of infiltrating CD11b-positive cells was much lower after treatment with caerulein. Immunostaining with F4/80, a marker of murine macrophages, confirmed that fewer macrophages were present in the pancreata of miR-21 −/− mice ( Fig. 2c,d ). Similarly, tissue sections stained with antibodies against Gr1, a neutrophil marker, showed less neutrophil infiltration in miR-21 −/− pancreata compared with WT mice ( Fig. 2e,f ). These data support the notion that miR-21 −/− mice have less-severe acute pancreatitis on caerulein treatment than WT mice. 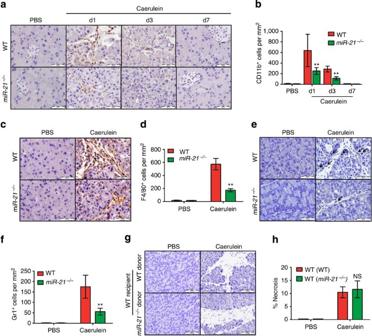Figure 2: Knockout ofmiR-21reduces inflammatory cell infiltrate to the pancreas during caerulein-induced pancreatitis. (a) Pancreata of WT andmiR-21−/−mice treated with caerulein were harvested at d1 (n=12), d3 (n=5) and d7 (n=5) after the last caerulein injection. Pancreatic sections were stained with anti-CD11b antibodies. (b) CD11b-positive cell counts in pancreatic tissue sections. (c) Pancreata of WT andmiR-21−/−mice treated with caerulein were harvested at d1 (n=12) after the last injection. Pancreatic sections were stained with antibodies against F4/80. (d) F4/80-positive cell counts in pancreatic tissue sections. (e) Pancreata of WT andmiR-21−/−mice treated with caerulein were harvested at d1 (n=12) after the last injection. Pancreatic sections were stained with antibodies against Gr1(Ly-6G). (f) Gr1-positive cell counts in pancreatic tissue sections. (g) Representative histological sections of pancreata stained with haematoxylin from caerulein-treated WT mice 5 weeks after transplantation with WT ormiR-21−/−bone marrow. Mice were euthanized 12 h after the last dose of caerulein. (h) Percentage of necrotic cells in pancreata. WT (WT), WT mice with WT bone marrow (n=5 for both PBS and treated groups); WT (miR-21−/−), WT mice withmiR-21−/−bone marrow (n=5 for both PBS and treated groups). Scale bars, 50 μm (a,c,e) and 100 μm (g). Values in bar graph are presented as mean±s.d. (n=5). **P<0.01 indicates a significant difference betweenmiR-21−/−tissues and the WT control (two-way analysis of variance). NS, not significant. Figure 2: Knockout of miR-21 reduces inflammatory cell infiltrate to the pancreas during caerulein-induced pancreatitis. ( a ) Pancreata of WT and miR-21 −/− mice treated with caerulein were harvested at d1 ( n =12), d3 ( n =5) and d7 ( n =5) after the last caerulein injection. Pancreatic sections were stained with anti-CD11b antibodies. ( b ) CD11b-positive cell counts in pancreatic tissue sections. ( c ) Pancreata of WT and miR-21 −/− mice treated with caerulein were harvested at d1 ( n =12) after the last injection. Pancreatic sections were stained with antibodies against F4/80. ( d ) F4/80-positive cell counts in pancreatic tissue sections. ( e ) Pancreata of WT and miR-21 −/− mice treated with caerulein were harvested at d1 ( n =12) after the last injection. Pancreatic sections were stained with antibodies against Gr1(Ly-6G). ( f ) Gr1-positive cell counts in pancreatic tissue sections. ( g ) Representative histological sections of pancreata stained with haematoxylin from caerulein-treated WT mice 5 weeks after transplantation with WT or miR-21 −/− bone marrow. Mice were euthanized 12 h after the last dose of caerulein. ( h ) Percentage of necrotic cells in pancreata. WT (WT), WT mice with WT bone marrow ( n =5 for both PBS and treated groups); WT ( miR-21 −/− ), WT mice with miR-21 −/− bone marrow ( n =5 for both PBS and treated groups). Scale bars, 50 μm ( a , c , e ) and 100 μm ( g ). Values in bar graph are presented as mean±s.d. ( n =5). ** P <0.01 indicates a significant difference between miR-21 −/− tissues and the WT control (two-way analysis of variance). NS, not significant. Full size image To determine whether the reduced severity of acute pancreatitis in miR-21 −/− mice was due to decreased macrophage activation, we profiled the pro-inflammatory gene expression in bone marrow-derived macrophages (BMDMs). Macrophages display remarkable plasticity and follow two distinct states of polarized activation: the classically activated (M1) phenotype and the alternatively activated (M2) phenotype [22] . On M1 stimuli such as lipopolysaccharides, macrophages secrete cytokines (including TNF-α, interleukin (IL)-1β and IL-6) and enzymes such as prostaglandin-endoperoxide synthase 2 (Ptgs2), to promote an inflammatory response. In response to the T-helper type 2 cytokines IL-4 and IL-13, M2 polarization of macrophages dampens inflammation and promotes tissue remodelling [22] . Studies of acute pancreatitis show an early and intense M1 activation of macrophages, characterized by high expression of TNF-α and other M1 genes [21] , [23] , [24] . When treated with lipopolysaccharides, only the levels of the chemokine Cxcl-9 and the enzyme gene Ptgs2 were lower in miR-21 −/− BMDMs compared with the WT BMDMs ( Supplementary Fig. 3a ). On the other hand, on IL-4 (an M2 stimulus) addition, expression of anti-inflammatory genes, such as Arg1 , Csf1 , Ccl22 and Ccl17 , was decreased by miR-21 deletion ( Supplementary Fig. 3b ). To test the relative role of miR-21 in bone marrow-derived inflammatory cells during pancreatitis, we performed bone marrow transplantation using WT mice (with CD45.1) as recipients and miR-21 −/− or WT mice (both with CD45.2) [25] as donors. Before bone marrow transplantation, we analysed peripheral blood lineage cells and found no differences in cell populations between WT and miR-21 −/− mice. At 4 weeks after bone marrow transplantation, mice were analysed for haematopoietic recovery and level of chimerism. Analysis of white blood cells in peripheral blood indicated normal haematopoietic recovery with no significant differences between mice transplanted with bone marrow isolated from WT or miR-21 −/− mice ( Supplementary Fig. 4 ). Flow cytometry analysis of peripheral blood mononuclear cells for the presence of donor-derived leukocytes expressing CD45.2 showed a high and equivalent level of chimerism in recipient mice (87.05±4.62% (mean±s.d.) in WT; 87.24±5.78% in miR-21 −/− ; n =8 in each group). Further analysis of peripheral blood lineage cells indicated a similar level of chimerism in granulocytes, B cells, T cells and monocytes ( Supplementary Figs 4 and 5 ). We then treated animals with caerulein at 5 weeks after transplantation. The response to caerulein-induced acute pancreatitis in WT mice receiving miR-21 −/− bone marrow was similar to that in WT mice transplanted with WT bone marrow ( Fig. 2g,h ). Collectively, these data suggest that the phenotypic difference in acute pancreatitis between caerulein-treated WT and miR-21 −/− mice is unlikely to be due to differences in macrophages or other bone marrow-derived blood cells, and more likely to depend on the intrinsic response of acinar cells. The expression of necroptosis genes and miR-21 targets The severity of experimental pancreatitis in rodents positively correlates with necroptosis but negatively with apoptosis [10] . In mice, necrosis is the major mechanism of acinar cell death in caerulein-induced acute pancreatitis [10] . We first determined whether deletion of miR-21 increases cell apoptosis in the pancreata at day 1 post treatment. In agreement with a previous report [10] , we found few apoptotic acinar cells as judged by terminal deoxynucleotidyl transferase nick end labelling (TUNEL) in the pancreata of WT mice, but based on cell morphology some inflammatory cell apoptosis was inferred ( Fig. 3a ). Yet, TUNEL staining of inflammatory cells and acinar cells in miR-21 −/− pancreata was elevated compared with the WT controls ( Fig. 3a,b ). We also measured cleaved caspase-3 using immunohistochemistry (IHC) and found more cells stained positively in tissues from miR-21 −/− mice than those from the WT controls ( Fig. 3c,d ). Next, we analysed the expression of RIP1, RIP3 and FADD in the pancreata of WT and miR-21 −/− mice, as these proteins are part of the necrosome that plays a key role in caerulein-induced pancreatitis. In line with previous observations [3] , RIP3 expression level was dramatically elevated in the pancreata of caerulein-treated WT mice; however, RIP3 levels in miR-21 −/− pancreata were significantly lower than in WT controls post treatment ( Fig. 3e ). In addition, FADD protein was lower in miR-21 −/− pancreata compared with WT controls. Levels of RIP1 were elevated by caerulein treatment in both WT and miR-21 −/− pancreata, yet miR-21 deletion produced little change ( Fig. 3e ). Lastly, we probed the expression of five reported miR-21 target genes ( PDCD4 , PTEN , SPRY2 , FASL and BCL-2 ). Only Pten and FasL expression was higher in miR-21 −/− mice than in WT mice (1.6- and 2.1-fold, respectively, Fig. 3f ). The expression of Pdcd4, Spry2 and Bcl-2 remained largely unchanged. These data indicate that miR-21-mediated target suppression may be effective for some but not all miR-21 gene targets in the pancreata. 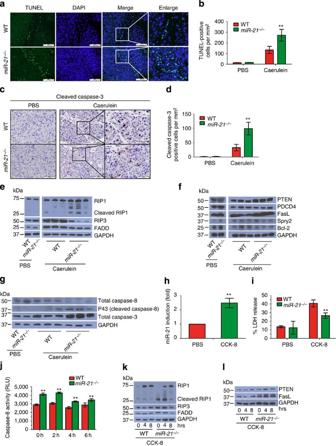Figure 3: Inhibition of acute pancreatitis inmiR-21−/−mice correlates with activation of caspase-8 and downregulation of RIP1, RIP3 and FADD through miR-21 targets in acinar cells. (a) TUNEL showing cellular apoptosis in pancreata from caerulein-treated WT andmiR-21−/−mice at d1 (n=12 per group) after the last dose of caerulein. Scale bars, 100 μm. (b) TUNEL-positive cell counts in pancreatic tissue sections (n=5 per group). (c) IHC of cleaved caspase 3. Pancreata of WT andmiR-21−/−mice treated with caerulein were harvested at d1 (n=12) after the last caerulein injection. Pancreatic sections were stained with antibodies against cleaved caspase 3. Scale bars, 100 μm, except in the enlarged area (far right). (d) Cleaved caspase-3-positive cell counts in pancreatic tissue sections. (e–g) Western blotting analyses of protein expression in pancreata. Pancreata of WT andmiR-21−/−mice treated with caerulein were harvested at d1 after the last dose (one animal per lane). (e) Expression of RIP1, RIP3 and FADD; (f) miR-21 targets; (g) expression of caspase-8 and caspase-3. Each blot was replicated three times. (h) Expression of miR-21 in acinar cells treated with supramaximal CCK-8. Acinar cells were isolated from WT andmiR-21−/−mice, and incubated for 8 h with CCK-8. Total RNA was extracted from acinar cells and miR-21 expression was quantified by real-time PCR. (i) Acinar cells were isolated from WT andmiR-21−/−mice, and incubated for 8 h with CCK-8. Cellular necrosis was determined by measuring LDH release. (j) Acinar cells were treated with CCK-8 for 2, 4 or 6 h, and then caspase-8 activity was measured using a luminescence assay normalized to GAPDH expression; RLU, relative luminescence units. (k,l) Western blotting analyses of protein expression in acinar cells treated with CCK-8. **P<0.01 indicates a significant difference between the indicated two groups (t-test inh; two-way analysis of variance in others). Figure 3: Inhibition of acute pancreatitis in miR-21 −/− mice correlates with activation of caspase-8 and downregulation of RIP1, RIP3 and FADD through miR-21 targets in acinar cells. ( a ) TUNEL showing cellular apoptosis in pancreata from caerulein-treated WT and miR-21 −/− mice at d1 ( n =12 per group) after the last dose of caerulein. Scale bars, 100 μm. ( b ) TUNEL-positive cell counts in pancreatic tissue sections ( n =5 per group). ( c ) IHC of cleaved caspase 3. Pancreata of WT and miR-21 −/− mice treated with caerulein were harvested at d1 ( n =12) after the last caerulein injection. Pancreatic sections were stained with antibodies against cleaved caspase 3. Scale bars, 100 μm, except in the enlarged area (far right). ( d ) Cleaved caspase-3-positive cell counts in pancreatic tissue sections. ( e – g ) Western blotting analyses of protein expression in pancreata. Pancreata of WT and miR-21 −/− mice treated with caerulein were harvested at d1 after the last dose (one animal per lane). ( e ) Expression of RIP1, RIP3 and FADD; ( f ) miR-21 targets; ( g ) expression of caspase-8 and caspase-3. Each blot was replicated three times. ( h ) Expression of miR-21 in acinar cells treated with supramaximal CCK-8. Acinar cells were isolated from WT and miR-21 −/− mice, and incubated for 8 h with CCK-8. Total RNA was extracted from acinar cells and miR-21 expression was quantified by real-time PCR. ( i ) Acinar cells were isolated from WT and miR-21 −/− mice, and incubated for 8 h with CCK-8. Cellular necrosis was determined by measuring LDH release. ( j ) Acinar cells were treated with CCK-8 for 2, 4 or 6 h, and then caspase-8 activity was measured using a luminescence assay normalized to GAPDH expression; RLU, relative luminescence units. ( k , l ) Western blotting analyses of protein expression in acinar cells treated with CCK-8. ** P <0.01 indicates a significant difference between the indicated two groups ( t -test in h ; two-way analysis of variance in others). Full size image Given the role of miR-21 targets in the extrinsic apoptosis pathway [3] , we hypothesized that upregulation of miR-21 targets in the pancreas elevates caspase-8 activity, which in turn downregulates RIP1 and RIP3 expression and acinar cell necrosis. Analysing caspase-8 activity, first we found that the expression of total caspase-8 was reduced in miR-21 −/− pancreata compared with WT controls post treatment, but the active form of caspase-8 (that is, cleaved caspase-8 protein (p43)) was upregulated in miR-21 −/− pancreata ( Fig. 3g ). The expression of a downstream caspase (total caspase-3) was significantly upregulated in miR-21 −/− pancreata, but no cleaved caspase-3 products were detected (data not shown). Next, we isolated acinar cells to recapitulate necrosis in vitro . miR-21 expression was higher in WT cells treated with cholecystokinin-8 (CCK-8), which stimulates necrosis in vitro ( Fig. 3h ). CCK-8 induced significant necrotic cell death, as judged by LDH activity (an indicator of mitochondrial rupture and necrosis), in WT acinar cells—an effect inhibited by miR-21 genetic ablation ( Fig. 3i ). Caspase-8 activity, however, was higher in miR-21 −/− acinar cells than in WT cells at the basal level and with CCK-8 induction ( Fig. 3j ). Four hours post CCK-8 treatment, RIP1 processing had significantly increased in miR-21 −/− acinar cells compared with WT controls ( Fig. 3k ), and Pten and FasL expression were elevated as well ( Fig. 3l ). These results support the possibility that miR-21 deficiency leads to less necrotic cell death and higher caspase-8 activity in isolated acinar cells and in the pancreata. To determine whether CCK receptor expression is affected by miR-21 genetic depletion, we measured the expression of CCK receptors A and B in pancreatic tissues from mice treated with caerulein, as well as in isolated acinar cells treated with CCK-8. We found no significant differences in CCK receptors A and B expression between WT and miR-21 −/− tissues ( Supplementary Fig. 6a ) or between isolated WT and miR-21 −/− cells ( Supplementary Fig. 6b ). In addition, we found that the amylase activity in the supernatant did not differ between WT and miR-21 −/− acinar cells treated with CCK-8 for 1–4 h ( Supplementary Fig. 6c ). These data indicate that miR-21 deficiency affects neither expression nor function of CCK receptors. The difference in serum amylase activities in Fig. 1g is likely to be due to the differential necrotic death rate of WT and knockout acinar cells in the pancreata. Caspase inhibition promotes necrosis in miR-21 −/− mice To test whether elevated caspase-8 activity is responsible for the seen protective effects of miR-21 deficiency against caerulein-induced acute pancreatitis, we pre-treated animals with z-VAD-fmk, a pan-caspase inhibitor. z-VAD-fmk pre-treatment significantly enhanced pancreatitis severity in miR-21 −/− mice as judged by morphology ( Supplementary Fig. 7a ) and histological scores for necrosis ( Supplementary Fig. 7b ). We also tested the efficacy of z-IETD-fmk, a caspase-8-specific inhibitor [26] , [27] , and similarly, z-IETD-fmk strongly sensitized miR-21 −/− mice to caerulein-induced pancreatitis ( Supplementary Fig. 7c,d ). In combination with our in-vitro data, these results indicate that the potential mechanism underlying the observed reduction in acute pancreatitis severity in miR-21 −/− mice can be attributed to the increased activity of caspase-8, an endogenous negative regulator of necroptosis. miR-21 deficiency attenuates L -Arg-induced pancreatitis As a high dose of L -Arg also induces acute necrotizing pancreatitis in rodents [28] , [29] and potentially in humans [30] , we employed this model to test whether the protective effect of miR-21 ablation was reproducible and model independent. Extensive pancreatic tissue injury was observed in WT mice 3 days after L -Arg treatment; yet, in miR-21 −/− mice pancreata were largely intact ( Supplementary Fig. 8a ). Serum amylase and lipase activity were significantly elevated in WT mice compared with miR-21 −/− mice. ( Supplementary Fig. 8b,c ). Histological analyses confirmed the reduced severity of acinar cell necrosis in miR-21 −/− mice compared with WT mice ( Supplementary Fig. 8d ). These data provide further evidence that genetic deletion of miR-21 protects pancreata from necrotic injury during acute pancreatitis. miR-21 inhibition in WT mice ameliorates acute pancreatitis Given the attenuation of acute pancreatitis in miR-21-deficient mice, we sought to determine whether inhibiting miR-21 with a locked nucleic acid (LNA)-based stable, nontoxic backbone-modified oligonucleotide complementary to miR-21 (anti-miR-21) could effectively treat or prevent caerulein-induced acute pancreatitis. In a treatment study to determine whether anti-miR-21 reverses ongoing acute pancreatitis, we injected anti-miR-21, 20 or 50 mg kg − 1 , into WT mice after the last dose of caerulein. Neither dose reduced disease severity. In a prevention study, we delivered anti-miR-21 simultaneously with caerulein into WT mice. Compared with either control anti-miR or vehicle (PBS), anti-miR-21 administration significantly downregulated miR-21 ( Fig. 4a ) and upregulated its targets Pten and FasL ( Fig. 4b ). Consistent with gene expression, acute pancreatitis severity was consistently attenuated by anti-miR-21 ( Fig. 4c–f ). These observations complement our findings that miR-21 deletion in mice protects the pancreas and indicate that prophylactic anti-miR-21 administration protects animals from caerulein-induced pancreatic injury. 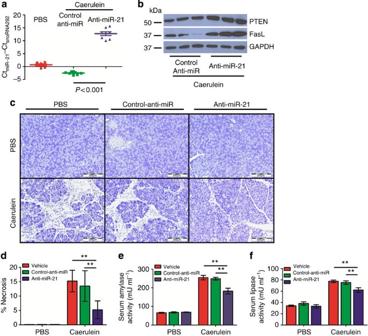Figure 4: Inhibition of miR-21in-vivoprotects mice from caerulein-induced pancreatitis. (a) Expression of miR-21 in caerulein-induced pancreatitis from WT mice injected with anti-miR-21 or a control (Control-anti-miR) (n=8 per group). Pancreatic tissues were harvested at d1 after the last injection. (b) Western blotting analyses of Pten and FasL expression in pancreata of treated WT mice at d1 after the last injection (one animal per lane). (c) Representative histological sections of WT mouse pancreata stained with haematoxylin at d1 after the last dose of caerulein. Scale bars, 200 μm. (d) Percentage of necrotic cells in pancreata. (e) Serum amylase activity in WT mice (n=8 per group) 6 h after the last injection. (f) Serum lipase activity in WT mice (n=8 per group) 6 h after the last injection. **P<0.01 indicates a significant difference between the indicated groups (one-way analysis of variance (ANOVA) inaand two-way ANOVA in others). Figure 4: Inhibition of miR-21 in-vivo protects mice from caerulein-induced pancreatitis. ( a ) Expression of miR-21 in caerulein-induced pancreatitis from WT mice injected with anti-miR-21 or a control (Control-anti-miR) ( n =8 per group). Pancreatic tissues were harvested at d1 after the last injection. ( b ) Western blotting analyses of Pten and FasL expression in pancreata of treated WT mice at d1 after the last injection (one animal per lane). ( c ) Representative histological sections of WT mouse pancreata stained with haematoxylin at d1 after the last dose of caerulein. Scale bars, 200 μm. ( d ) Percentage of necrotic cells in pancreata. ( e ) Serum amylase activity in WT mice ( n =8 per group) 6 h after the last injection. ( f ) Serum lipase activity in WT mice ( n =8 per group) 6 h after the last injection. ** P <0.01 indicates a significant difference between the indicated groups (one-way analysis of variance (ANOVA) in a and two-way ANOVA in others). Full size image miR-21-deficient mice are protected from TNF-α-induced shock A common complication of acute pancreatitis is a systemic inflammatory response syndrome (SIRS), which often leads to multiple organ failure. RIP1- and RIP3-mediated cellular necroptosis drives mortality during TNF-α-induced SIRS [31] . We hypothesized that miR-21 deletion protects against lethal SIRS. We administered TNF-α to mice, to test the role of miR-21 in TNF-α-induced SIRS. We first evaluated animal survival using a lethal TNF-α injection. All WT mice died within 10 h, whereas only 10% of miR-21 −/− mice succumbed; 20% of miR-21 −/− mice eventually survived TNF-α shock ( P <0.0001, n =10 per group, log-rank test, Fig. 5a ). We then examined systemic changes at 3 h after TNF-α injection in a separate set of mice. The serum LDH levels were significantly reduced in miR-21 −/− mice compared with WT controls ( Fig. 5b ). The ileum, kidney and liver were collected and tissue damage was evaluated by histological analyses. We found that villi were more swollen and inflammatory infiltrates were greater in the ileum of WT than that of miR-21 −/− mice ( Fig. 5c,d ). Moderately increased kidney tubule dilatation, degeneration and necrosis were also found in WT compared with miR-21 −/− mice ( Fig. 5e,f ). Liver damage was slightly inhibited in miR-21 −/− mice compared with WT mice, but the difference was not statistically significant ( Fig. 5g,h ). These data demonstrate that loss of miR-21 protects mice from TNF-α-induced tissue damage and mortality. 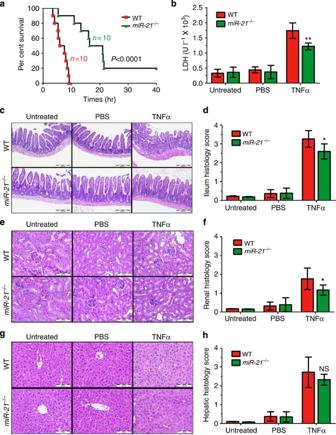Figure 5: miR-21 deletion protects mice from TNF-α-induced shock. (a) Survival of WT andmiR-21−/−mice challenged with 9 μg TNF-α (n=10 per group,P<0.0001). (b) Serum samples of WT andmiR-21−/−mice were collected 3 h after challenge with 9 μg TNF-α and LDH activities were analysed (n=5 per group, a separate cohort). Representative histological sections of the ileum (c), kidney (e) and liver (g) stained with haematoxylin and eosin 3 h after TNF-α injection in WT andmiR-21−/−mice. Scale bars, 200 μm for the ileum and 100 μm for the kidney and liver. (n=5 for each group). The tissue damage score for the ileum (d), kidney (f) and liver (h) was evaluated. *P<0.05 and **P<0.01 indicate a significant difference between WT andmiR-21−/−mice treated with TNF-α (two-way analysis of variance). NS, not significant. Figure 5: miR-21 deletion protects mice from TNF-α-induced shock. ( a ) Survival of WT and miR-21 −/− mice challenged with 9 μg TNF-α ( n =10 per group, P <0.0001). ( b ) Serum samples of WT and miR-21 −/− mice were collected 3 h after challenge with 9 μg TNF-α and LDH activities were analysed ( n =5 per group, a separate cohort). Representative histological sections of the ileum ( c ), kidney ( e ) and liver ( g ) stained with haematoxylin and eosin 3 h after TNF-α injection in WT and miR-21 −/− mice. Scale bars, 200 μm for the ileum and 100 μm for the kidney and liver. ( n =5 for each group). The tissue damage score for the ileum ( d ), kidney ( f ) and liver ( h ) was evaluated. * P <0.05 and ** P <0.01 indicate a significant difference between WT and miR-21 −/− mice treated with TNF-α (two-way analysis of variance). NS, not significant. Full size image Fas/FasL and necrostatin-1 treatment in pancreatitis The pathological aggravation of acute pancreatitis is reported to be related to the Fas/FasL pathway. First, FasL expression in pancreatic tissues from mice treated with caerulein was consistently lower than that from sham-treated animals [32] . Second, in patients with acute pancreatitis, FasL serum levels decreased significantly as acute pancreatitis severity increased [33] . Third, Fas deficiency exacerbates caerulein-induced pancreatitis [34] . To determine whether FasL, a miR-21 target, is responsible for the observed protection exerted by miR-21 deletion in caerulein-induced pancreatitis, we treated WT mice with caerulein plus recombinant mouse FasL (mFasL), finding that mFasL did not significantly influence pancreas injury ( Supplementary Fig. 9a,b ). We then applied MFL3, a FasL-inhibiting antibody, in caerulein-treated miR-21 −/− mice. We found that MFL3 did not affect the severity of pancreatitis in miR-21 −/− mice ( Supplementary Fig. 9c,d ). As controls, we also administered MFL3 to WT mice and mFasL to miR-21 −/− mice treated with caerulein and found no significant impact. We next sought to inhibit necroptosis using necrostatin-1 (Nec-1) in both caerulein-induced pancreatitis and TNF-α-induced shock in WT and miR-21 −/− mice. Nec-1 is an allosteric inhibitor of RIPK1 kinase activity and thus is a potential drug candidate against pathologic necroptosis. In the acute pancreatitis model, we found Nec-1 exacerbates pancreas damage in WT mice, which is in line with the published data [35] . Yet, Nec-1 had no effect on miR-21 −/− mice treated with caerulein ( Supplementary Fig. 10a,b ). In the TNF-α-induced shock model, we found that Nec-1 protected against liver damage moderately in WT or miR-21 −/− mice treated with TNF-α, but not against ileum damage; kidney damage was increased significantly by Nec-1 in both WT and miR-21 −/− mice ( Supplementary Fig. 11a–f ). These experiments indicate that the blockade of necroptosis with Nec-1, as a drug candidate, did not adequately protect against acute pancreatitis or septic shock-induced tissue damage. Nonetheless, these results in combination with genetic ( Fig. 1 ) and pharmacologic data with anti-miR-21 ( Fig. 4 ) suggest that inhibiting miR-21, rather than Nec-1 treatment or Fas/FasL manipulation, is effective in ameliorating tissue damage in acute pancreatitis induced by caerulein. miR-21 in recruitment of the necrotic complex To delineate the molecular mechanism of miR-21 in necrosis, we examined necrotic cell death using mouse embryonic fibroblasts (MEFs) as an in-vitro cell model. In MEFs and many other cells, the combination of TNF-α and cycloheximide (TC) induces apoptosis, whereas the addition of z-VAD-fmk to this regimen (TCZ) promotes necrosis [36] . We found that on TCZ treatment, miR-21 −/− MEFs exhibited less necrosis than WT cells; no differences in apoptosis were observed ( Fig. 6a–d ). The recruitment of RIP1 and RIP3 to FADD is essential to form the necrosome, which is required for necroptosis. Immunoprecipitation (IP) experiments with anti-FADD antibodies revealed that after treatment with TCZ, significantly less RIP1 and RIP3 protein was associated with FADD in miR-21 −/− MEFs compared with WT MEFs ( Fig. 6e ). We then determined the role of miR-21 target genes ( Pten and FasL ) in cellular necrosis of miR-21 −/− MEFs treated with TCZ. Notably, these two miR-21 targets were upregulated in miR-21 −/− MEFs [15] , in miR-21 −/− pancreata ( Fig. 3c ) and in miR-21 −/− acinar cells ( Fig. 3i ). Knockdown of either Pten or FasL via small interfering RNA (siRNA; Fig. 6f ) significantly enhanced cellular death of TCZ-treated miR-21 −/− MEFs ( Fig. 6g ). As expected, recruitment of RIP1 and RIP3 to FADD increased when Pten or FasL expression was downregulated ( Fig. 6h ). These data indicate that upregulation of Pten and FasL is partially responsible for the reduced necrosis observed in cells and animals without miR-21. 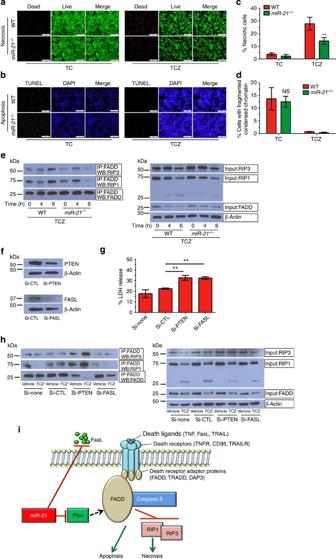Figure 6: The effects of miR-21 target genes on necrosis in MEFs. (a) Cell viability of WT andmiR-21−/−MEFs treated with TC or TCZ. To detect live and dead cells, cells were stained with Calcein AM (green, live cells) and ethidium homodimer-1 (red, dead cells) 6 h after treatment. (b) Apoptotic cell death of WT andmiR-21−/−MEFs treated with TC or TCZ. To assess apoptosis, cells were stained with TUNEL (green, apoptotic cells) and DAPI (4’, 6-diamidino-2-phenylindole; blue, nucleus). Scale bars, 200 μm. (c) Bar graph shows the percentage of necrotic cells ina. (d) Bar graph shows the percentage of cells with fragmented condensed chromatin inb. (e) Formation of the FADD-RIP1-RIP3 complex in WT andmiR-21−/−MEFs measured by FADD co-IP. (f) Western blotting shows the efficacy of siRNA knockdown inmiR-21−/−MEFs transfected with siRNA-PTEN or siRNA-FASL. (g) Bar graph shows the percentage of necrotic cells using the LDH assay after TCZ treatment and siRNA transfection. (h) Formation of the FADD-RIP1-RIP3 complex with the introduction of siRNA againstPTENandFASLinmiR-21−/−MEFs. Cells were treated with TCZ as indicated. The formation of FADD-RIP1-RIP3 complex was measured by FADD co-IP inmiR-21−/−MEFs with siRNA-PTEN and siRNA-FASL. **P<0.01 indicates a significant difference between the marked two groups (two-way analysis of variance (ANOVA) incandd, and one-way ANOVA ing). NS, not significant. (i) Schematic representation shows the proposed regulation of the necrotic complex by miR-21 via suppression of FasL and Pten. Figure 6: The effects of miR-21 target genes on necrosis in MEFs. ( a ) Cell viability of WT and miR-21 −/− MEFs treated with TC or TCZ. To detect live and dead cells, cells were stained with Calcein AM (green, live cells) and ethidium homodimer-1 (red, dead cells) 6 h after treatment. ( b ) Apoptotic cell death of WT and miR-21 −/− MEFs treated with TC or TCZ. To assess apoptosis, cells were stained with TUNEL (green, apoptotic cells) and DAPI (4’, 6-diamidino-2-phenylindole; blue, nucleus). Scale bars, 200 μm. ( c ) Bar graph shows the percentage of necrotic cells in a . ( d ) Bar graph shows the percentage of cells with fragmented condensed chromatin in b . ( e ) Formation of the FADD-RIP1-RIP3 complex in WT and miR-21 −/− MEFs measured by FADD co-IP. ( f ) Western blotting shows the efficacy of siRNA knockdown in miR-21 −/− MEFs transfected with siRNA-PTEN or siRNA-FASL. ( g ) Bar graph shows the percentage of necrotic cells using the LDH assay after TCZ treatment and siRNA transfection. ( h ) Formation of the FADD-RIP1-RIP3 complex with the introduction of siRNA against PTEN and FASL in miR-21 −/− MEFs. Cells were treated with TCZ as indicated. The formation of FADD-RIP1-RIP3 complex was measured by FADD co-IP in miR-21 −/− MEFs with siRNA-PTEN and siRNA-FASL. ** P <0.01 indicates a significant difference between the marked two groups (two-way analysis of variance (ANOVA) in c and d , and one-way ANOVA in g ). NS, not significant. ( i ) Schematic representation shows the proposed regulation of the necrotic complex by miR-21 via suppression of FasL and Pten. Full size image Recent studies have identified new participants in regulated necrosis [1] , [2] , [37] ; yet, the role of noncoding RNAs in necroptosis and pancreatitis remains unexplored. The major finding of this study is that miR-21 regulates necrotic cell death, and that deletion of miR-21 prevents necroptosis during caerulein-induced acute pancreatitis. In mouse models of acute pancreatitis, acinar cell death is regarded as a form of regulated necrosis, specifically necroptosis that depends on the activity of two kinases, RIP1 and RIP3 (refs 3 , 4 ). As miR-21 is overexpressed in the pancreata from mice treated with caerulein, we examined the potential pathological function of miR-21 in acute pancreatitis. Compared with WT animals, miR-21 −/− mice are protected against acinar cell necrosis and oedema, demonstrating, for the first time, a novel pathogenic contribution of miR-21 in this acute pancreatitis model. Moreover, this result was validated in a second model of acute pancreatitis induced by L -Arg. Acute pancreatitis is the most common reason for hospitalization due to gastrointestinal disease. Necrosis is the final cause of pancreatic tissue injury during acute pancreatitis and it precipitates several major pathobiologic processes such as pancreatic inflammation and oedema, and leads to systemic involvement of extrapancreatic organs [17] . We demonstrate that miR-21 inhibition using LNA-based oligonucleotides also protects mice from caerulein-induced pancreas injury. Given the paucity of treatment options for acute pancreatitis, inhibition of miR-21 may be a feasible therapeutic strategy against acute pancreatitis and its secondary clinical complications. To dissect the mechanism of miR-21 action, we reasoned that the reduced severity of acute pancreatitis in miR-21-deficient mice could be due to less cell death caused by acinar cell necrosis, a limited pro-inflammatory response, or a combination of both processes. The bone marrow transplantation experiment provided evidence to exclude the possibility that inflammatory infiltration by macrophages or other leukocytes played a differential role in the less-severe acute pancreatitis phenotype in miR-21 −/− mice. Thus, although we appreciate that inflammatory cells are essential for caerulein-induced pancreatitis injury in mice, our data indicate that the necrotic death of acinar cells is probably the predominant underlying cause of the phenotypic difference between miR-21 −/− and WT mice. This role for miR-21 was further confirmed in isolated acinar cells independent of the presence of inflammatory cells. When treated with CCK-8 as an in-vitro stimulus of necrosis, miR-21-deficient acinar cells displayed less necrotic cell death than CCK-8-treated WT cells. Similar protection was observed in primary miR-21 −/− MEFs undergoing stimulated necrosis. Notably, we found that miR-21 plays opposite roles in two forms of cell death— miR-21 −/− MEF cells display reduced necrotic cell death, but are more susceptible to apoptotic cell death stimulated by DNA damage [14] , [15] . We further distinguished the mechanism of miR-21 in necroptosis by examining the expression of RIP1, RIP3, FADD and caspase-8 in the pancreata of miR-21 −/− mice. Caerulein treatment elevates pancreatic RIP3 protein levels, yet miR-21 deletion significantly reduces the induction of this critical component of necroptosis. The expression of two endogenous inhibitors of necrosis—FADD and caspase-8—are differentially affected. FADD is moderately downregulated, yet the activated form of caspase-8 is significantly upregulated by miR-21 deletion. We reasoned that elevated caspase-8 activity is probably insufficient to induce massive apoptosis but may be adequate to inhibit RIP3 expression and reduce necroptosis. We tested this hypothesis by pretreating miR-21 −/− mice with z-VAD-fmk (a pan-caspase inhibitor) or z-IETD-fmk (a caspase-8-specific inhibitor), which largely abolished the protective effect of miR-21 genetic ablation on acute pancreatitis. These data suggest that elevated caspase-8 activity is pivotal in protecting against acute pancreatitis mediated by miR-21 deficiency. This is consistent with previous reports showing that deletion of caspase-8 elevates necroptosis [6] , [7] . The precise mechanism by which caspase-8 is engaged to prevent necroptosis without triggering apoptosis in acinar cells during acute pancreatitis remains elusive. miR-21 participates in the regulation of multiple gene networks and it has been reported to directly repress the expression of more than 30 genes [38] . These genes include FasL and Pten , which are involved in death receptor-mediated extrinsic apoptosis pathways [38] ( Fig. 6i ). FasL is a type II transmembrane protein that belongs to the TNF family and induces necroptosis through a complex consisting of caspase-8 and FADD by binding its cognate receptor CD95 (ref. 1 ). It is reported that Pten promotes TNF-α- or FasL-induced apoptosis by facilitating caspase-8 activation that depends on FADD [25] , [39] . We found that FasL and Pten are upregulated in miR-21 −/− pancreata and thus we examined whether modulation of these miR-21 targets affects necrotic cell death. Both necrotic cell death and necrosome recruitment were enhanced in miR-21 −/− cells under necrotic stimuli when the expression of FasL or Pten was knocked down. Yet, manipulating FasL alone cannot recapitulate the phenotype of protecting mice from caerulein-induced acute pancreatitis as does miR-21 genetic deletion or inhibition with anti-miR-21. These findings suggest that miR-21 modulates cell necroptosis through negative regulation of FasL and Pten, and most probably many other targets, and further supports a key role for miR-21 in a complex network of interrelated death receptor-mediated apoptosis and necroptosis ( Fig. 6i ). Taken together, our data support the idea that miR-21 is a pro-necroptosis miRNA. In future studies, it will be critical to determine how miR-21 enhances RIP1/3-mediated necroptosis and thereby creates a pro-inflammatory microenvironment with a strong necrosis element contributing to many other life-threatening conditions. Murine pancreatitis models The miR-21 knockout mouse line ( miR-21 −/− ) [15] was crossed back to the C57BL/6J genetic background through speed congenic breeding. Female mice (22–25 g, age 7–8 weeks) were used for caerulein-induced pancreatitis and male mice were used for the bone marrow transplantation and L -arg-induced pancreatitis models. We did not find sex bias in caerulein-induced acute pancreatitis in mice. Mice, randomized by body weight if there are two or more groups, were administered two series of 8-hourly intraperitoneal (i.p.) injections (separated by 40 h) of a supramaximally stimulating dose of caerulein (50 μg per kg body weight, Sigma-Aldrich, St Louis, MO). The final day of caerulein injection was defined as day 0 (d0). For the mechanistic studies of necroptosis, z-VAD-fmk or z-IETD-fmk (BD Pharmingen, San Jose, CA) was dissolved in dimethyl sulfoxide at 10 mg ml − 1 and administered i.p. 15 min before the first dose of caerulein at 5 mg kg − 1 (ref. 40 ). For the L -Arg model, mice were injected (i.p.) with L -Arg hydrochloride (8%, pH 7.0 in PBS) in two doses of 4 g kg − 1 , 1 h apart; animals were euthanized after 72 h [28] . No lethality was observed. All animal experiments were performed under protocols approved by the University of Louisville Institutional Animal Care and Use Committee and in accordance with the Guide for the Care and Use of Laboratory Animals (NIH). To determine the water content, pancreata were obtained at 12 h after the last caerulein injection and the wet tissue weight determined. Tissues were then freeze dried overnight and reweighed to obtain a dry weight; pancreatic water content was calculated as the difference between the wet and dry tissue weights, and was expressed as a percentage of the total (wet) weight. TNF-α-induced SIRS model Recombinant mouse TNF-α (Shenandoah Biotechnology, Warwick, PA) was injected intravenously via the tail vein into WT and miR-21 −/− mice in a volume of 0.2 ml (9 μg in endotoxin-free PBS); animals were observed hourly for survival. In a separate set of experiments, mice were killed 3 h after TNF-α injection, and serum and tissue samples of the ileum, kidney and liver were collected. Histopathology of tissue damage of the ileum, kidney and liver were evaluated by a pathologist in a double-blind manner, on paraffin sections on a scale ranging from 0 (completely unaffected tissue), 1 (negligible damage), 2 (minor damage), 3 (moderate damage) to 4 (severe damage). Histology and apoptosis Pancreatic tissues were collected and fixed overnight in 10% neutral-buffered formalin. Fixed tissue was paraffin embedded, sectioned (5 μm thick) and stained with haematoxylin for morphological analyses. Quantification of histological scoring for acute pancreatitis and necrotic death of acinar cells was performed as described [41] . Cells with swollen cytoplasm, loss of plasma membrane integrity and leakage of organelles into interstitium were considered necrotic. The necrotic areas were automatically calculated based on haematoxylin staining for pancreas or haematoxylin and eosin staining for other tissues using Olympus cellSens software [42] . The extent of acinar cell necrosis was expressed as the per cent of the total acinar tissue that was occupied by necrotic areas, meeting the criteria for necrosis: (i) the presence of acinar cell ghosts or (ii) vacuolization and swelling of acinar cells and the destruction of the histoarchitecture of whole or parts of the acini. For IHC, primary antibodies against CD11b, F4/80 (Abcam, Cambridge, MA) and Gr1 (BD Pharmingen, San Diego, CA) were used to assess inflammatory cell infiltration. Deparaffinized and rehydrated sections were boiled in Na-citrate buffer (10 mM, pH 6.0) for 10 min for antigen retrieval. Tissue sections were developed using the Ultra Vision Detection System, anti-rabbit (Thermo Scientific). About 1,500 positive cells were counted per slide per animal ( n =5 animals in each group), to calculate the percentage of positively stained cells. For immunofluorescence staining of amylase, pancreatic tissue sections were incubated with anti-α-amylase antibody (1:400, Sigma) for 2 h at room temperature. After being rinsed with PBS, the sections were incubated with Alexa Fluor-488 goat anti-rabbit (1:100, Invitrogen, Carlsbad, CA) for 1 h at room temperature. After another PBS rinse, the sections were incubated with 1.0 μg ml − 1 4′, 6-diamidino-2-phenylindole for 5 min. Slides were analysed under fluorescence microscopy. Morphometry of amylase density was based on computer-aided area measurement of amylase protein expression (excluding islets). For the TUNEL assay to detect apoptosis, deparaffinized pancreatic sections were incubated with 20 μg ml − 1 protease K for 15 min at room temperature, then washed with PBS and incubated with the TUNEL reaction mixture (Roche Applied Science) for 60 min at 37 °C in a humidified atmosphere. Tissue sections were incubated with converter peroxidase (with anti-fluorescein antibody) and subsequently with the 3, 3′-diaminobenzidine substrate. Images were acquired using an Olympus IX51 microscope and the cellSens digital imaging software. Nuclei with condensed or fragmented chromatin (brown cells) were considered apoptotic; 2,000 acinar cells were counted per slide per animal ( n =5 animals in each group). We also performed IHC staining for cleaved caspase-3 as condensed fragmented chromatin is not specific [43] . Mouse primary cell preparation Acinar cells were prepared by collagenase digestion following an established protocol [44] . Briefly, mice were fasted overnight and the pancreas was removed, minced and washed with PBS with 0.01% soybean trypsin inhibitor (Sigma-Aldrich). Tissues were rinsed with Ham’s F12K medium (Invitrogen) with antibiotics and 0.1 mg ml − 1 soybean trypsin inhibitor, 5 mg ml − 1 BSA faction V (Sigma-Aldrich) and 10% fetal bovine serum. The mixture was centrifuged at 500 g for 2 min and the pellet was resuspended in 10 ml digestive solution containing 200 U ml − 1 collagenase type III (Sigma-Aldrich) and 0.2 mg ml − 1 BSA fraction V. Digestions were performed at 37 °C with shaking at 130 cycles per min for 30 min. The pellet was then collected by centrifugation at 500 g for 2 min, resuspended and passed through a pipette several times. Large cell blocks were removed by filtration through a 70-μm cell strainer. The filtered cells were washed twice with Ham’s F12K medium. Acinar cells obtained were maintained in Ham’s F12K supplemented with 10% fetal bovine serum, 0.1 mg ml − 1 soybean trypsin inhibitor and 5 mg ml − 1 BSA faction V, and incubated at 37 °C with 5% CO 2 . To stimulate necrosis, acinar cells were treated with CCK-8 (100 nmol l − 1 ) for 2–8 h [45] . MEFs were prepared according to an established protocol [15] , [46] . Primary WT and miR-21 −/− MEFs were treated with TNF-α (T, 20 ng ml − 1 ), cycloheximide (C, 1 μg ml − 1 ) and/or z-VAD-fmk (Z, 20 μM). BMDMs were prepared using an established protocol [47] . Mice (8 weeks old) were killed and hind legs were removed. All muscle tissues from the bones were removed using scissors. The femur was separated and flushed with PBS using a 3-ml syringe and a 23-gauge needle. Bone marrow was passed through a pipette several times to make a single-cell suspension. Cells were washed with PBS twice before being plated onto a culture dish. Cells were maintained in DMEM supplemented with 10% fetal bovine serum and 10 ng ml − 1 murine granulocyte macrophage colony-stimulating factor (R&D Systems, Minneapolis, MN), and incubated at 37 °C with 5% CO 2 . Enzyme activity and necrosis Blood was collected from mice through the tail vein and kept at 4 °C for 1 h before centrifugation at 4,000 g for 20 min at 4 °C. Serum was collected from the supernatant and amylase activity was measured by using EnzyChrom α-Amylase assay kit (BioAssay Systems, Hayward, CA), according to the manufacturer’s protocol. Lipase activity was assayed using the Lipase Detection Kit (Colorimetric) (ab102524, Abcam). Caspase-8 activity was measured by homogeneous luminescent assay using the Caspase-Glo 8 kit (Promega, Madison, WI), according to the manufacturer’s protocols. For MPO activity, lung samples were homogenized in 20 mM phosphate buffer (pH 7.4) and the pellet was resuspendend in 50 mM phosphate buffer (pH 6.0) containing 0.5% hexadecyltrimethylammonium bromide (Sigma). The suspension was sonicated for 30 s, centrifuged at 10,000 g for 5 min and the supernatant was used for the MPO assay. The supernatant was mixed with 1.6 mM tetramethylbenzidine (Sigma), 80 mM sodium phosphate buffer (pH 5.4) and 0.3 mM hydrogen peroxide. This mixture was then incubated at 37 °C for 110 s, the reaction was terminated with 0.18 M H 2 SO 4 and the absorbance was measured at 450 nm. This absorbance was then corrected for the calculated dry weight of the tissue samples. Cellular necrosis was determined by measuring LDH with a cytotoxicity assay kit (Promega), according to the manufacturer’s protocols. Dead cells were also visualized using the LIVE/DEAD Viability/Cytotoxicity kit (Invitrogen). Briefly, cells were cultured on sterile glass coverslips and treated with cytotoxic agents. After the indicated treatment time, cells were washed with PBS and then stained with 2 μM calcein-AM and 4 μM ethidium homodimer-1. After incubation for 30 min at room temperature, cells were washed with PBS and viewed under fluorescence microscopy. At least 1,500 positive-staining cells were counted per slide per animal ( n = 5 animals in each group), to calculate the percentage of the labelled cells. RNA preparation and quantitative PCR To measure M1 and M2 expression in BMDM, BMDM were isolated from WT and miR-21 −/− mice, and total RNA was extracted using Trizol (Invitrogen) and run on an Agilent Bioanalyzer 2100, to ensure an A260/A280 ratio in the range of 1.8–2.2 and an rRNA ratio (28S/18S)>0.9. RNA was reverse-transcribed with the iScript Reverse Transcription Supermix kit (BIO-RAD, Hercules, CA). Real-time PCR was performed using the iQ SYBR Green Supermix (BIO-RAD) and CFX96 Real-Tme PCR system (BIO-RAD), with primers designed based on Universal Probe Library (Roche) with ACTB as the reference (oligonucleotide sequences were provided in Supplementary Table 1 ). Bone marrow transplantation Twelve-week-old recipient WT CD45.1 mice (B6.SJL- Ptprc a Pep3 b /BoyJ; Jackson Laboratory, Bar Harbor, Maine; n =16) were conditioned with 950 cGy total body irradiation from a caesium source (Gamma-cell 40; Nordion, Ontario, Canada). At 24 h after irradiation, the mice were transplanted with bone marrow cells (1 × 10 7 cells per mouse in 0.1 ml PBS) isolated from tibias and femurs of 11-week-old CD45.2 WT and miR-21 −/− donor mice, through the retro-orbital plexus with a 27-gauge needle. Six mice received WT bone marrow and ten received miR-21 −/− bone marrow. After 4 weeks, recipient mice were characterized for haematopoietic recovery and chimerism by determining the relative percentages of CD45.2 cells in peripheral blood. Co-staining with markers of T cells (CD3), B cells (B220), granulocytes (Gr-1) and monocytes (CD11b) was used to determine the level of chimerism in lineage-specific cells. Peripheral blood was obtained through retro-orbital bleeding for whole blood cell counts using a HemaVet 950 system (Drew Scientific Group, Oxford, CT) and nucleated cells were analysed by flow cytometry (LSRII, BD Biosciences), to determine the percentage of CD45.2 cells. Both the recipient and donor mice were maintained on normal chow throughout the experiment. RNA interference and miR-21 inhibition Low-passage MEFs were transfected with 25 nM siRNA duplexes targeting PTEN and FASL by using Lipofectamine RNAiMAX reagent. After 48 h, the cells were collected and assayed to ensure silencing was achieved. siRNA duplex oligonucleotides, purchased from Dharmacon (Lafayette, CO), were: FASL (5′- UACCAGUGCUGACCAUUUA -3′), PTEN (5′- GAUCAGCAUUCACAAAUUA -3′) and a control (Non Targeting siRNA Pool 2). For miR-21 inhibition in cells, the Ambion Anti-miR miRNA Inhibitors (Life Technologies, Grand Island, NY) were used with the Negative Control 1 as the control for transfection and cells were collected after 48 h. For miR-21 inhibition in murine acute pancreatitis, LNA-modified antisense to miR-21 (anti-miR-21) was mixed with caerulein and i.p. injected into mice. The control (control-anti-miR) was the miRCURY LNA miRNA inhibitor control Negative Control A (Exiqon, Woburn, MA) and it has no more than 70% homology to any sequence in the mouse genome. The total dose for anti-miR-21 or control-anti-miR is 20 mg kg − 1 of body weight. Western blot analyses and IP Pancreatic tissues, acinar cells and MEFs cells were lysed with radio-IP assay buffer (Cell Signaling, Boston, MA) supplemented with protease inhibitor (Calbiochem, Billerica, MA). Soluble proteins were subjected to SDS–PAGE before transferring to polyvinylidene difluoride membranes. The following antibodies were used: RIP3 (ab58828, 1:200), Spry2 (ab50317, 1:2,400), FasL (ab68338, 1:500), all Abcam; and RIP1 (D94C12, 1:1,000), caspase-8 (4927, 1:1,000), cleaved caspase-8 (8592, 1:1,000), GAPDH (14C10, 1:1,000), Pdcd4 (D29C6, 1:1,000), FADD (ab124812, 1:1,000), Bcl-2(50E3, 1:1,000) and Pten (D4.3, 1:1,000), all from Cell Signaling. β-Actin (1:5,000) primary antibody was purchased from Sigma. IP was performed by using the Pierce Classic IP Kit, according to the manufacturer’s protocols. Briefly, 1 × 10 6 MEFs were cultured in 10 cm petri dishes and treated with TCZ for the indicated times. Cells were then lysed with radio-IP assay buffer and soluble proteins were incubated with 2 μg anti-FADD antibody (M-19, Santa Cruz) overnight at 4 °C. After incubation, the antibody and lysate mixture was supplemented with protein A/G plus agarose and incubated for 1 h. The immunoprecipitates were washed for four times with IP lysis and wash buffer, and eluted by boiling the agarose beads in elution buffer. Samples were subjected into SDS–PAGE before western blotting and uncropped scans of all blot images were provided in Supplementary Fig. 12 . Statistical analysis Data are presented as mean with s.d. The SPSS16.0 software (SPSS Inc. Chicago, IL) was used for all statistical analyses. An unpaired two-tailed Student’s t -test was performed for two-group comparisons. One-way analysis of variance was performed for multiple group comparisons with one independent variable and two-way analysis of variance for multiple group comparisons with two independent variables ( miR-21 gene status, treatment, histology and so on). For the survival analysis, Kaplan–Meier results were analysed by log-rank test. Statistical significance was set at * P <0.05 or ** P <0.01. How to cite this article: Ma, X. et al . The oncogenic microRNA miR-21 promotes regulated necrosis in mice. Nat. Commun. 6:7151 doi: 10.1038/ncomms8151 (2015).